Graphitic nanostripes in silicon carbide surfaces created by swift heavy ion irradiation The controlled creation of defects in silicon carbide represents a major challenge. A well-known and efficient tool for defect creation in dielectric materials is the irradiation with swift ( E kin ≥500 keV/amu) heavy ions, which deposit a significant amount of their kinetic energy into the electronic system. However, in the case of silicon carbide, a significant defect creation by individual ions could hitherto not be achieved. Here we present experimental evidence that silicon carbide surfaces can be modified by individual swift heavy ions with an energy well below the proposed threshold if the irradiation takes place under oblique angles. Depending on the angle of incidence, these grooves can span several hundreds of nanometres. We show that our experimental data are fully compatible with the assumption that each ion induces the sublimation of silicon atoms along its trajectory, resulting in narrow graphitic grooves in the silicon carbide matrix. Silicon carbide (SiC) is an important material because of its unusual thermal, mechanical and electronic properties. It is used as a biocompatible substrate [2] , in nuclear [3] and novel electronic applications [4] , [5] , [6] , and more recently has attracted a lot of attention as a substrate for the growth of epitaxial graphene [7] , [8] , [9] , [10] , [11] and quasi-free standing graphene [12] , [13] . In addition, SiC exhibits a plethora of defect-related phenomena. For example, Bockstedte et al. [14] reported many-body effects in the excitation spectrum of a defect in SiC, defect-induced magnetism in neutron-irradiated 6H-SiC single crystals was found [15] , and it was demonstrated that a Si vacancy in SiC could serve as a quantum system for a single-photon source [16] . Most recently, it was suggested to use room temperature coherent spin alignment of silicon vacancies in 4H- and 6H-SiC for spintronic applications, quantum information processing as well as magnetometry [17] . So the question arises how efficient defect engineering can be accomplished in SiC, a material that is known for its superior resistance even in environments with high levels of ionizing particle radiation, as, for example, in fission reactors or in space. It is well known in the materials science community that swift heavy ions (SHI) with kinetic energies of 100 MeV or more can be used to study materials under extreme conditions, which can otherwise not be achieved [18] , [19] , [20] , [21] . The main reason for these unique properties of SHI is the intense electronic excitation (expressed in terms of electronic energy loss or stopping power, S e =d E /d x ) that is induced in the solid by the projectile along its trajectory. This initial energy deposition dissipates in a series of complex processes giving rise to structural modifications, depending on the physical properties of the target material. These modifications range from isolated point defects to complete phase transitions. Corresponding irradiation experiments on SiC revealed that a significant displacement of atoms in SiC can only be obtained by electronic excitation if the energy deposition is S e ≥34 keV per nm [22] , which is unachievable with monoatomic projectiles. Thus, in the electronic stopping regime, irradiation with d E /d x below this threshold will induce only isolated point defects. Depending on the fluence, these point defects can accumulate but this will still not give rise to complete amorphization of the material [23] . Instead, it has been observed that even a recrystallization of the defective structure may occur. This damage recovery has been attributed to the competing effects due to nuclear collisions and electronic excitations [23] , [24] , [25] . These findings however impose a severe limitation on SHI irradiation as a tool for defect engineering of SiC. In this paper, we present clear evidence that this limitation is not valid for the surface of SiC single crystals. Our experiments under grazing incidence show that even individual ions produce extended permanent defects in the form of graphitic grooves at stopping powers as low as S e =17 keV per nm; our calculations even predict a threshold of S e =7 keV per nm. Furthermore, we have identified a novel effect in the thermal dissipation process, which is relevant for the correct description of the groove length in glancing angle SHI irradiation experiments. We show that it is neither necessary to overcome the extremely high decomposition temperature of SiC of 3,010 K, nor is defect accumulation required for the groove creation. Instead, the defect formation mechanism is due to a thermal process similar to the one used nowadays for graphene production. Because both, groove density and groove length, can be adjusted by simply changing the ion beam parameters, our results are valuable for defect engineering of SiC surfaces. Irradiation As samples we used Si-terminated 6H-SiC wafers (Pam-Xianmen) cleaned with isopropyl alcohol. For the irradiation, two different experiments were performed at the IRRSUD beamline of the GANIL, one with a stopping power of S e =17 keV per nm (81 MeV Ta 24+ , fluence of 1 × 10 9 ions per cm 2 ) at an angle of Θ=1.1° and the other with S e =22 keV per nm (117 MeV Pb 31+ , fluence of 1 × 10 9 ions per cm 2 ) at angles of Θ=0.6–4.2°. The angle Θ is measured with respect to the surface plane. To achieve this high precision, the targets were mounted on a vertical target holder, which can be rotated around the vertical axis by a stepping motor implemented in the irradiation chamber. This stepping motor has (together with its gear) a stepping width of about 0.02°. The repeatability of the motor is better than 0.1°, describing the relative uncertainty between two angles measured in the same experiment. The overall error bar for the incidence angle was found to be below 0.2° (see Methods). Topography Atomic force microscopy (AFM) images taken after irradiation in air reveal for both ions extended but shallow depressions on the surface running along the ion beam direction as can be seen in Fig. 1a . The constant width of ≈20 nm and depth of ≈2 Å suggest that the ion-induced damage affects only the topmost layer of atoms. To further investigate the nature of these surface modifications, the grooves were imaged in ultra-high vacuum (UHV) in a non-contact mode [25] with compensation of electrostatic forces. We find that groove length varies as a function of incidence as can readily be seen from Fig. 1a,b . By analysing a number of samples where the angle of incidence Θ was varied, we find the result shown in Fig. 1d , that is, the groove length increases significantly with decreasing angle of incidence. The statistical error bars of the experimental data are mostly due to the beam divergence (≤0.2°) and the statistical nature of the stopping process. The data points roughly follow the relation L = d /tan(Θ), the best fit yields d =6.3 nm. This relation follows from a simple geometrical model, where L is the measured groove length in the SiC surface and d is a constant that corresponds to the maximum depth from which SHI-related damage can still be detected at the surface (see Fig. 1a and ref. 26 ). Note that at smaller angles we find a significant deviation, which will be discussed below. 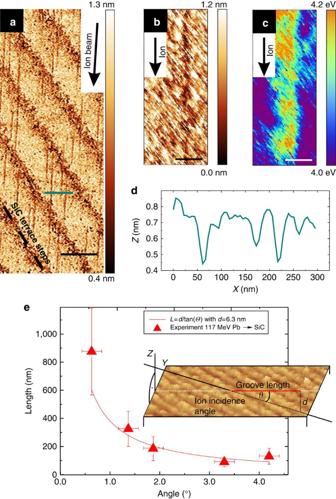Figure 1: Graphitic grooves due to ion irradiation. (a) AFM (tapping mode) images of irradiated 6H-SiC single crystal (81 MeV Ta, Θ=1.1°, fluence 10 ions per μm2; scale bar, 400 nm). Line scan reveals their typical depths and widths. Grooves are perfectly aligned with the direction of the incoming ion beam, marked with the white arrow. (b) Non-contact mode image taken in UHV (81 MeV Ta, Θ=1.5°; scale bar, 40 nm). (c) Simultaneously recorded KPFM image shows that the grooves have a higher work function difference than the surrounding undamaged SiC (scale bar, 40 nm). The work function determined from this data is consistent with a graphitic groove. (d) Topographic lineprofile corresponding to the marked line ina. (e) Measured groove length as a function of angle of incidence (117 MeV Pb red triangles). Red line depicts the best fit to the 117 MeV Pb data using the relationL=d/tan(Θ) withd=6.3 nm; inset shows the corresponding geometry. Figure 1: Graphitic grooves due to ion irradiation. ( a ) AFM (tapping mode) images of irradiated 6H-SiC single crystal (81 MeV Ta, Θ=1.1°, fluence 10 ions per μm 2 ; scale bar, 400 nm). Line scan reveals their typical depths and widths. Grooves are perfectly aligned with the direction of the incoming ion beam, marked with the white arrow. ( b ) Non-contact mode image taken in UHV (81 MeV Ta, Θ=1.5°; scale bar, 40 nm). ( c ) Simultaneously recorded KPFM image shows that the grooves have a higher work function difference than the surrounding undamaged SiC (scale bar, 40 nm). The work function determined from this data is consistent with a graphitic groove. ( d ) Topographic lineprofile corresponding to the marked line in a . ( e ) Measured groove length as a function of angle of incidence (117 MeV Pb red triangles). Red line depicts the best fit to the 117 MeV Pb data using the relation L = d /tan(Θ) with d =6.3 nm; inset shows the corresponding geometry. Full size image Surface potential The grooves on the SiC surface are unambiguously related to the irradiation. The measured depth of the grooves is fully compatible with a region of atoms missing from the topmost layer. To determine what kind of atoms are at the bottom of the grooves, we performed quantitative Kelvin probe force microscopy (KPFM) to measure the local work function [27] , [28] . We used ultra-thin layers of graphite that were mechanically exfoliated onto the SiC sample to calibrate the unknown work function of the tip. On these graphite and graphene flakes, we measure a local contact potential that we attribute to the work function of graphite and graphene [29] , [30] , namely, 4.65 and 4.5 eV (ref. 28 ), respectively. The ion-induced grooves can be clearly seen in the KPFM image (see Fig. 1c ) and their work function is higher than the work function of undamaged SiC. This shift upwards means that the work function in the region of the grooves has changed from the value of SiC, that is, 4.0 eV, towards the value one would expect for graphite or graphene (4.65–4.5 eV). This is in full agreement with the topography data if we assume that the topmost Si atoms are missing and the bottom of the grooves is rich in carbon. The absolute value of the observed shift is smaller than that one would expect for extended samples. But this kind of data is always limited by the spatial resolution of the KPFM method [31] , which is 100 nm in our case and thus much larger than the groove width. The direction of the shift towards graphite however suggests that the grooves are graphitic in nature. Etching To exclude the possibility that the surface was contaminated by an oxide and that the grooves were formed in SiO x instead of SiC, the irradiated samples were etched with hydrofluoridic acid for 10 min. Then, they were imaged again by AFM, see Fig. 2 . After etching, steps on the SiC appear sharp and straight, proving that the etch has worked. The grooves are however still there, telling us that they were indeed formed in the SiC surface itself and not in an oxide surface layer. 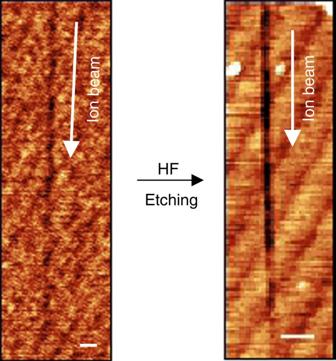Figure 2: Graphitic grooves remain after etching. AFM images of the irradiated (81 MeV Ta, Θ=1.5°) sample surface before (left image; scale bar, 40 nm) and after (right image; scale bar, 40 nm) etching in hydrofluoric acid. The grooves (direction of the beam marked with the white arrow) remain visible after the etch. Figure 2: Graphitic grooves remain after etching. AFM images of the irradiated (81 MeV Ta, Θ=1.5°) sample surface before (left image; scale bar, 40 nm) and after (right image; scale bar, 40 nm) etching in hydrofluoric acid. The grooves (direction of the beam marked with the white arrow) remain visible after the etch. Full size image The ion irradiation-induced damage we observe in SiC clearly differs from the modifications observed in other dielectrics (for example, Al 2 O 3 , SrTiO 3 , TiO 2 , SiO 2 , CaF 2 , polymethylmethacrylate) that have been irradiated under similar conditions [17] , [32] , [33] , [34] , [35] . In those materials, the surface typically shows elongated protrusions (or chains of protruding hillocks) aligned along the ion beam direction. In case of SrTiO 3 , these have been successfully interpreted as the remnants of a molten zone [18] , originating from a rapidly quenched thermal spike [36] induced by the ion. Here we observe missing material (grooves) instead of protruding molten material and in the following section we present an explanation why SiC behaves so differently. From the KPFM data and from the fact that the grooves exhibit a constant depth of ≈2 Å as can be seen in the AFM measurement in Fig. 1 , we deduce that the missing atoms are mostly surface Si atoms resulting in the formation of the groove. The preferential ejection of surface Si atoms suggests that the projectile triggers a temperature rise along the trajectory, which is sufficient to reach the Si sublimation temperature. Exactly this sublimation process makes the growth of epitaxial graphene on SiC single crystals at T =1,400 K possible [37] . If sublimation is of relevance in our case, it would indeed not be necessary to reach the decomposition temperature of 3,010 K to create a groove in SiC, but instead a much lower temperature and thus an energy deposition well below the proposed threshold of 34 keV per nm would suffice. The exact sublimation temperature for the conditions in an ion track, where a quenching of the thermal spike occurs on a time scale of about a few picoseconds, is unknown. In the following, we assume it to be T sub =1,900 K (for details see Supplementary Methods ). Note that in the volume, this mechanism would however not be relevant, as Si atoms cannot evaporate from a heated zone surrounded by an intact crystal lattice. This is the reason for the constant trench depth observed in our data. To test whether the origin of this modification is indeed connected to sublimation, the resulting lattice temperatures can be calculated with the two-temperature model (TTM) [38] , [39] , [40] . The TTM is a contiuum model based on two coupled heat diffusion equations for the electron and phonon system, respectively. The region where the temperature rise leads to a permanent modification is commonly called a ‘track’, which is assumed to manifest itself as a groove on the surface in our case. The TTM model has to be adapted here to take into account that the process takes place in close vicinity to the surface, thus breaking the cylindrical symmetry used in conventional TTM calculations. Therefore, the code we use here is based on a fully three-dimensional (3D) version of the TTM (equations 1 and 2). It was originally developed by us to describe so-called surface tracks in SrTiO 3 and to predict the respective stopping power threshold [26] . Here, it was further modified to accommodate a larger part of the beam–target interaction volume so that the influence of the surface can be studied in full detail. The TTM reads: Where the subscripts e and p refer to electron and phonon quantities. is the temperature, while C ( T ) and κ ( T ) are the heat capacity and thermal conductivity, respectively. The electron–phonon coupling parameter g controls the transfer of energy from the electrons to the phonons. Finally, is the energy deposition of the ions. Because SHI show no angular scattering, that is, their trajectory is a straight line and for every point of the ion trajectory, the actual energy deposition may be calculated using the following formula [41] The stopping power S e is obtained using the SRIM code, G ( t ) is a Gaussian with a half-width of 1 fs [41] and is the spatial electron distribution given by Waligorski et al. [42] For each point ( x 0 , y 0 , z 0 ) on the ion trajectory, the vector is oriented perpendicular to the ion beam axis. Finally, b is a normalization constant, so that The temperature-dependent phononic heat capacity C p ( T p ) and thermal conductivity κ p ( T p ) are taken from the literature [43] , [44] . Furthermore, we follow the commonly accepted concept that electrons in the conduction band of a dielectric behave like electrons in metals [45] . Thus, we assume that the electronic heat capacity C e ( T e ) can be described using the free-electron gas formalism, so that Here, the Fermi temperature T F is given by ħ is the Planck constant, m e the electron mass, k B is the Boltzmann constant and n e is the (free) electron density in the conduction band. The electron density effectively enters as a free parameter. While n e may be calculated explicitly using a kinetic approach like a Monte Carlo simulation [46] , such calculations are not feasible at the glancing incidence geometry considered here. Thus, as an estimation we use n e = ρ / A =4.8 × 10 22 cm −3 , where ρ and A are the density and mass of SiC. The electron–phonon coupling strength is difficult to determine. Experimentally, this quantity may be obtained by evaluating ablation rates [47] , measuring the thermoreflectance [48] or optical reflection [49] . However, these experiments are often performed at low laser intensities, which are not comparable to the SHI irradiation scenario. Moreover, to the best of our knowledge, no such data exist for dielectric materials. The electron–phonon coupling will in general depend explicitly on the electron distribution function, and therefore on the electron density, the electron temperature and so on [36] , [50] , [51] and thus on the specific excitation profile, that is, the laser pulse duration or like in this particular case, on the SHI energy. One often employed approximation is to treat the electron–phonon coupling parameter g as a constant, which is adopted in the present calculations (see equations 1 and 2). To determine the value of g , we fitted the calculated groove length to the experimentally measured ones (see below and Supplementary Methods for further details). From this fitting, we find g =4 × 10 18 J s −1 m −3 K −1 . This value is close to the value of g =6 × 10 18 J s −1 m −3 K −1 , which can be derived from ref. 52 . To calculate the lattice temperature resulting from SHI irradiation with the TTM, we can exploit the fact that the travelled length (projected onto the surface) of the ion beam with respect to its actual depth d perpendicular to the surface is given by L = d /tan(Θ). Thus, to calculate T p for irradiation with ions at an angle of Θ=1.9°, a simulation box with a length of x =400 nm, a width of y =40 nm and a depth of z =20 nm is required to accomodate the ion beam. Note that electrons leaving the vicinity of the track region are not considered here, as they do not contribute to the track formation. Then, equations 1 and 2 are solved on a (400 × 40 × 20) nm 3 grid using the finite difference method. The simulation box is surrounded by a thermal bath, while Neumann boundary conditions are used for the surface. While emission of phonons into the vacuum may be neglected, electrons with energies above the work function of SiC [53] can escape the surface. To account for this electron emission, we remove electrons at the surface with sufficient energies. Finally, it should be noted here that for the sake of simplicity, holes are completely neglected. The groove length is determined by measuring the extension of the surface region, which reaches the sublimation temperature of T sub =1,900 K, while the impact point of the ion is chosen as x =100 nm, y =0 nm, z =0 nm, where z =0 nm denotes the surface (see Fig. 3 ). As an example, we present the results for an irradiation with 117 MeV Pb ions at Θ=1.9°. The results for 400 fs and 1.5 ps after the ion impact can be seen in Fig. 3a,c . The area enclosed by the solid contour line in the surface plane ( x – y -plane, bottom left) is at T sub ≥1,900 K. Note that the decomposition temperature of 3,010 K is hardly reached and only in a very small region. 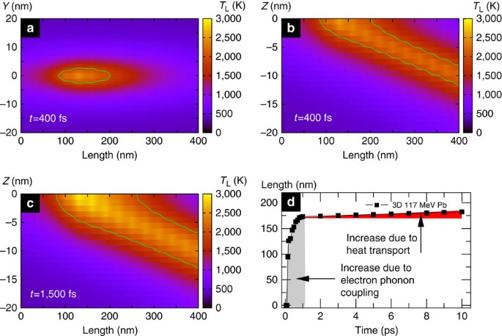Figure 3: Temperature profiles after ion impact. Three-dimensional TTM calculation for irradiation of SiC with 117 MeV Pb at Θ=1.9° at 400 fs (a) topview, (b) sideview and (c) 1.5 ps after the ion impact. (d) Heat is still transported at times when the temperature gradient between electronic and lattice temperature has already vanished. Figure 3: Temperature profiles after ion impact. Three-dimensional TTM calculation for irradiation of SiC with 117 MeV Pb at Θ=1.9° at 400 fs ( a ) topview, ( b ) sideview and ( c ) 1.5 ps after the ion impact. ( d ) Heat is still transported at times when the temperature gradient between electronic and lattice temperature has already vanished. Full size image Owing to the electron–phonon coupling, the track length evolves with time (length increase marked in Fig. 3d ) and reaches a length of 174 nm at 900 fs after the ion impact. At this time, the electron and lattice temperatures are roughly in equilibrium, that is, the energy transfer to the lattice described by equation 2 has stopped. However, the track length still increases at least up to 6 ps (see Fig. 3d , track length increase marked in red) as the energy is transported outwards, away from the trajectory. Because the track is located close to the surface, this leads to a notable effect: at Θ=1.9°, the increase in length is about 4%, that is, a maximum length of 180 nm is achieved. Note that this effect is exclusively due to the presence of the surface. The surface cannot dissipate heat except via irradiation, which is rather ineffective compared with the heat transport in bulk material via diffusion. In Fig. 3c , another effect can be observed: the extension of the heated zone is no longer symmetric with respect to the track but it is anisotropic now. The heated zone bulges outwards and extends further into the x direction. Thus, the projected track length is larger than it would be without the presence of the surface. To quantify the influence of the surface in more detail, we have calculated the track length with a conventional 1D TTM calculation, that is, assuming cylindrical symmetry. Here the calculation is done for perpendicular incidence and the resulting track is then tilted by the corresponding angle of incidence Θ. In Fig. 4 , the calculated values from the 1D model (solid line), the 3D model (squares) and the experimental data (triangles) are shown in comparison. Within the 1D TTM, the resulting lattice temperature is determined from the intersection of a cylinder (the ion track) with the surface. Thus, by tilting the ion beam (corresponding to the angle of incidence), the intersection of the cylinder with the surface becomes an ellipse, where the axis of the ellipse can be identified with the length and the width of the groove on the surface. Please note that this procedure is obsolete in our 3D description of the TTM. Here, the length and the width of the groove is readily obtained, as is shown in Fig. 3 . 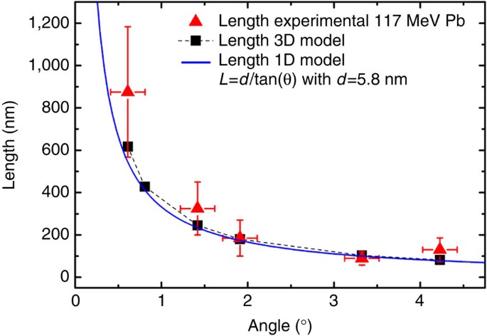Figure 4: Influence of the surface on heat transport. Comparison of calculated (blue line 1D; black squares 3D; dashed line to guide the eye) and experimental data (red triangles). Difference at small angles between 1D and 3D is due to the surface affecting the heat transport. Figure 4: Influence of the surface on heat transport. Comparison of calculated (blue line 1D; black squares 3D; dashed line to guide the eye) and experimental data (red triangles). Difference at small angles between 1D and 3D is due to the surface affecting the heat transport. Full size image In case of a 1D calculation, the groove length simply obeys the geometrical relation L = d /tan(Θ), where the value of d is identified as the groove diameter obtained from the 1D calculation. We find d =5.8 nm, which is slightly different from the best fit to the experimental data in Fig. 1 . The 3D groove lengths are always longer and the maximum difference of 13% is found at around Θ=0.6°. Note that, although the effect is discussed here quantitatively, its true significance will depend on the specific material properties, such as the thermal conductivity. Nevertheless, from this comparison, it is obvious that the surface plays a major role for the groove length. Because energy is transported easily in the surface plane and into the volume, but not across the surface into the vacuum, the groove is elongated. The track length shown in Fig. 4 (black squares) is thus a combination of two surface-induced effects: anisotropic heat transport and prolonged heat transport. Those effects will be large for materials where the transition temperature is low and the melting temperature is high. It should also be strongly pronounced in materials with excellent heat transport properties. In principle, both models give a satisfying agreement with the data, supporting the hypotheses that the ion indeed induces a thermal process at the surface, which gives rise to Si sublimation. However, the agreement with the 3D model is superior, especially in the case of extremely glancing angles. At these small angles, the predicted groove lengths in the 1D model are much too short and are only just within the experimental error bar. Our experimental data and the good agreement with the TTM results are strong points in favour of our hypothesis that a thermal process is responsible for the defect creation. However, the fact that also the 3D model underestimates the groove length may be an indication for additional, yet unidentified processes. In agreement with the negligible stopping cross-section in our energy regime, we rule out nuclear stopping, because we observe neither collision cascades nor signs of angular deflection in our experimental data. However, especially at the surface, many other mechanisms can contribute and have been shown to be important. The dissipation of energy from the electronic system to the lattice will have a more pronounced effect on the surface atoms, simply because mechanical constraints are less severe. This can even be exploited for surface nanostructuring with slow highly charged ions [54] and has also been observed for SHI. For example, in the case of Al 2 O 3 , hillocks are formed at the surface after irradiation with an electronic stopping power below the threshold for amorphous latent track production [32] . In this case, the authors proposed Coulomb explosion [55] , [56] as a possible mechanism. Other possibilities that have been discussed include electronic sputtering [57] and nanoscale viscous flow, but also microexplosions and shock waves caused by the thermal spike [58] , [59] , as well as increased surface damage by coherent displacement of lattice atoms [60] . In most cases, one would indeed expect a combination of mechanisms to be the origin for any kind of surface damage. Thus, it would certainly be of interest to compare our TTM data with, for example, molecular dynamics simulations or to measure the kinetic energy and angular distribution of the ejected particles to unravel the interplay as well as the respective contributions of the various defect creation mechanisms. This is however beyond the scope of the present paper. Given the good agreement between the 3D model and the experiments, we were encouraged to determine the so-called damage threshold, that is, the minimum energy necessary to induce these modifications. For this purpose, track lengths for various Pb ion energies are calculated. From Fig. 5 it can be seen that tracks start to appear at an ion energy of around 20 MeV. Thus, the damage threshold for grooves in SiC is found to be 20 MeV for Pb ions, which corresponds to a stopping power of around 7 keV per nm. This value is comparable to the one found earlier for surface tracks in SrTiO 3 (ref. 26 ) and can be obtained not only with monoatomic projectiles but also with ion beams from smaller accelerators. Experiments are underway to test this prediction of the theory. 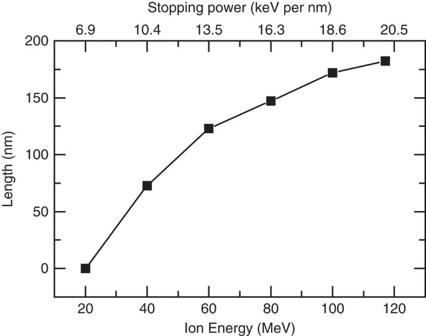Figure 5: Threshold for groove creation. Calculated track length for different Pb ion energies at Θ=1.9°. Numbers indicate the stopping power in keV per nm. Grooves can be created with a minimum ion energy of 20 MeV, corresponding to a stopping power of7 keV per nm. Figure 5: Threshold for groove creation. Calculated track length for different Pb ion energies at Θ=1.9°. Numbers indicate the stopping power in keV per nm. Grooves can be created with a minimum ion energy of 20 MeV, corresponding to a stopping power of 7 keV per nm. Full size image In summary, we have shown that in contrast to earlier bulk irradiation results, SiC sustains extended defects by individual SHI with moderate stopping power. From our data analysis we propose that due to the ion-induced electronic excitation and the subsequent thermal processes, Si sublimates from the surface into the vacuum along the trajectory, leaving a narrow carbon-rich groove behind. In addition, we have identified the surface as the origin of a new prolonged and anisotropic thermal heating process, which we could correctly describe with a 3D TTM model. The novel defect creation mechanism presented in our paper can be applied for defect engineering of SiC surfaces, as it has been recently demonstrated for SiC/graphene heterostructures, for example [28] . The nanostripes could also easily be used for techniques such as template-directed adsorption. Furthermore, our approach might be extended to create graphene nanoribbons with a controllable length and width, embedded in a SiC matrix, which would have great potential for applications [61] . Scanning probe microscopy The length of the surface grooves due to SHI irradiation was evaluated by AFM in tapping mode using a Veeco Dimension 3100 system. As probes, standard Si cantilever NCHR (Nanosensors, Neuchatel-Switzerland) were used. To get accurate measurements of the length, the scan frame was kept smaller than 3 × 3 μm 2 . Additional SPM characterization was performed in UHV ( p base =2 × 10 −10 mbar) using a RHK UHV 7500 system with PLL Pro 2 controller. Simultaneously with non-contact AFM measurements, KPFM measurements were performed using the built-in lock-in amplifier of the PLL Pro 2. For this, Si Vistaprobe T300 cantilevers (Nanoscience instruments, Phoenix, USA) were employed. During the frequency modulation KPFM measurements, an AC voltage of U AC =1 V with f AC =1 kHZ was applied to the tip. The resulting electrostatic force was minimized by an additional U DC , which corresponds to the local contact potential difference between tip and surface. Etching The sample was treated by sequential ultrasonic baths in acetone, methanol and isopropyl alcohol (p.a., VWR Prolabo). This was followed by a cleaning step in hot piranha solution (3:1 mixture of 96% sulphuric acid (Suprapur, Merck) and 30% hydrogen peroxide (p.a., AppliChem)). Subsequently, the sample was rinsed with deionized water (18 Ωcm; Millipore) and dried in a stream of high-purity argon (5.0, Air Liquide). For HF etching, the sample was placed in a 10% HF solution (made from p.a. 40% HF; Fluka) for 10 min, then cleaned by an ultrasonic bath in deionized water and finally dried in a stream of high-purity argon. Simulation As discussed in the paper, the evaluation of the groove length is performed in such a way that the length of the area, where the lattice temperature exceeds the sublimation temperature T sub , is extracted from the simulations. Obviously, the choice of the sublimation temperature directly determines the groove length. Another key parameter that directly determines the groove length is the value of the electron–phonon coupling paramter g . In this study, it is found that a sublimation temperature of around T sub =1,900 K and an electron–phonon coupling parameter of g =4 × 10 18 J s −1 m 3 K −1 give the best agreement with our experimental data. For details see Supplementary Methods . Calibration of angle of incidence This relative error was obtained by the following procedure: the motor was moved to its zero position, a fixed position inherent to the motor assembly. Afterwards, the motor was moved to an arbitrary angle, and returned to its zero position. Any difference in the display at the two zero-point positions is due to the repeatability of the motor. To obtain the absolute zero-degree orientation, a telescope was mounted on the optical axis of the beamline. The position at which the sample surface (seen through the telescope) is parallel to this direction was determined as zero degree and is accurate within 0.2°. This procedure was repeated for every experimental run. To further ensure correct irradiation conditions, we applied the following procedure [62] : if we assume an efficiency of unity (every ion creates a groove), we can calibrate the angle of incidence, because during an experiment the fluence is fixed and scales with the sine of Θ. How to cite this article : Ochedowski, O. et al. Graphitic nanostripes in silicon carbide surfaces created by swift heavy-ion irradiation. Nat. Commun. 5:3913 doi: 10.1038/ncomms4913 (2014).